Nanomotor lithography The rapid miniaturization of devices and machines has fuelled the evolution of advanced fabrication techniques. However, the complexity and high cost of the state-of-the-art high-resolution lithographic systems are prompting unconventional routes for nanoscale patterning. Inspired by natural nanomachines, synthetic nanomotors have recently demonstrated remarkable performance and functionality. Here we report a new nano-patterning approach, named ‘nanomotor lithography’, which translates the autonomous movement trajectories of nanomotors into controlled surface features. As a proof of principle, we use metallic nanowire motors as mobile nanomasks and Janus sphere motors as near-field nanolenses to manipulate light beams for generating a myriad of nanoscale features through modular nanomotor design. The complex spatially defined nanofeatures using these dynamic nanoscale optical elements can be achieved through organized assembly and remote guidance of multiple nanomotors. Such ability to transform predetermined paths of moving nanomachines to defined surface patterns provides a unique nanofabrication platform for creating diverse nanodevices. A variety of lithographic techniques are now available for direct processing of materials at the nanoscale [1] , [2] , [3] . While the resolution of these techniques has continued to improve, the cost of their implementation and system complexity have also increased substantially. For example, traditional photolithographic nanofabrication techniques rely on costly masks [4] , while electron and focused ion beam writing require expensive beam sources and elaborate control systems [5] , [6] . Similarly, sophisticated equipment is required for lithographic techniques based on scanning probes and optical tweezers [7] , [8] , [9] , [10] . Alternate strategies, involving self-assembling nanostructures, have been explored to improve the versatility and lower the fabrication costs [11] , [12] , [13] , [14] , [15] , [16] . However, arbitrary direct writing cannot be performed by these methods due to the lack of mobility of these nano components. Inspired by natural biological systems [17] , [18] , the recent development of synthetic nanomotors has paved the way towards major advances in nanoscience [19] , [20] , [21] , [22] , [23] , [24] , [25] . These self-propelled nanoscale devices can convert various energies into autonomous movement and overcome miniaturization challenges governed by force-scaling laws. Like their natural counterparts, these versatile man-made nanomotors have demonstrated advanced capabilities, including precise speed regulation and spatial motion control, along with self-organization and collective movement for a wide range of practical applications [26] , [27] , [28] , [29] , [30] . The advanced performance of such self-propelled nanomotor systems can address the challenges encountered with existing nano-patterning techniques and lead to powerful tools for direct surface writing at the nanoscale level. We report here a new versatile and cost-effective direct-write nano-patterning methodology, named ‘nanomotor lithography’ (NML), using nanomotors that ‘swim’ over photoresist surfaces for creating spatially defined complex surface patterns. This approach is made possible by developing an ‘on-the-fly’ strategy for manipulating the light incident on the moving nanomotors. Self-propelled metallic nanowire motors and Janus sphere motors with distinct optical properties are used here as the moving optical elements. Once light reaches the moving nanomotors, they can effectively perform near-field lithography: the opaque metallic nanowire motors allow for the nanoscale blocking of light while the transparent Janus sphere motors allow for efficient near-field concentration of light. Using such a versatile method, various nanoscale features are generated through modular nanomotor design. Due to the small dimension of the nanowire motors and the near-field focusing effect of the Janus sphere motors, sub-wavelength resolution can be achieved. The self-propelled motion along with magnetically guided control makes the new nanomotor approach simple, cost-effective and obviates the requirements of elaborate control systems used in common surface patterning techniques. Spatially defined nanofeatures are obtained by remote magnetic guidance of the nanomotors, while parallel writings are achieved through organized assembly and controlled motion of multiple nanomotors. This transformative combination preserves the high spatial resolution of near-field optical lithography while gaining the ability to control the patterns in a predefined and parallel manner, creating a unified tool for constructing and studying nanomaterials and nanodevices. 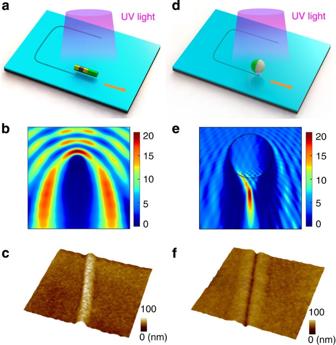Figure 1: Nanomotor lithography. (a) Schematic of nanomotor lithography by using a nanowire motor as a self-propelled nanomask. (b) FDTD model of the intensity of light blocking by a 200-nm-diameter Pt nanowire in water (refraction indexn=1.34). The plane shown is parallel to the light propagation direction. Wavelength of light, 400 nm. The black circle represents the cross-section of the nanowire. (c) Atomic force microscopy (AFM) topographical three-dimensional (3D) patterns of a ridge-line feature created by a 200-nm-diameter wire nanomotor swimming in a 1% H2O2solution. (d) Schematic of nanomotor lithography by using a Janus sphere motor as a self-propelled nanolens. (e) FDTD model of the intensity of light passing through a 2.16-μm-diameter Janus sphere (n=1.62 for polystyrene) in water (n=1.34). The black circle represents the contour of the sphere and the right hemisphere is coated with a 10-nm Pt film. (f) AFM topographical 3D pattern of a trench line feature created by a 2.16-μm-diameter Janus sphere motor swimming in a 5% H2O2solution. Both 3D perspective images incandfare shown with displayed areas of 6 × 6 μm2. Description of NML Figure 1 illustrates the basic concepts of NML using the self-propelled metallic nanowire motors as nanomasks ( Fig. 1a–c ) and Janus sphere motors as near-field nanolenses ( Fig. 1d–f ). In the first case, a motile, remote-controlled metallic nanowire motor replaces the traditional photomask and acts as a dynamic nanoscale optical element that locally shields the photoresist beneath it from ultraviolet exposure, and hence generates a surface pattern that mirrors its moving trajectory due to a lower exposure dosage over the predetermined guided path ( Fig. 1a ). After development, the directional trajectories of the nanomotors will be revealed on the polymer surface as raised ridge lines. The Au/Ni/Au/Pt four-segment nanowire motor ‘masks’, fabricated by a template-assisted electrochemical deposition protocol, are self-propelled over the photoresist surface by self-electrophoresis in the presence of H 2 O 2 fuel [19] , [20] , [21] . Finite-difference time-domain (FDTD) numerical simulation of such localized light blocking is displayed in Fig. 1b , while the nanofeature created by a stationary nanowire photomask is shown in Supplementary Fig. 1 . The atomic force microscopy (AFM) image of Fig. 1c displays a ridge line created by a 200-nm-diameter nanowire motor swimming with a speed of 15 μm s −1 . The width of the ridge line (measured as full-width at half maximum (FWHM)) is ~300 nm, demonstrating a successful autonomous patterning of a feature smaller than the wavelength (400 nm) of incident light. Figure 1: Nanomotor lithography. ( a ) Schematic of nanomotor lithography by using a nanowire motor as a self-propelled nanomask. ( b ) FDTD model of the intensity of light blocking by a 200-nm-diameter Pt nanowire in water (refraction index n =1.34). The plane shown is parallel to the light propagation direction. Wavelength of light, 400 nm. The black circle represents the cross-section of the nanowire. ( c ) Atomic force microscopy (AFM) topographical three-dimensional (3D) patterns of a ridge-line feature created by a 200-nm-diameter wire nanomotor swimming in a 1% H 2 O 2 solution. ( d ) Schematic of nanomotor lithography by using a Janus sphere motor as a self-propelled nanolens. ( e ) FDTD model of the intensity of light passing through a 2.16-μm-diameter Janus sphere ( n =1.62 for polystyrene) in water ( n =1.34). The black circle represents the contour of the sphere and the right hemisphere is coated with a 10-nm Pt film. ( f ) AFM topographical 3D pattern of a trench line feature created by a 2.16-μm-diameter Janus sphere motor swimming in a 5% H 2 O 2 solution. Both 3D perspective images in c and f are shown with displayed areas of 6 × 6 μm 2 . Full size image In the second case, NML relies on Janus sphere motors as near-field nanolenses ( Fig. 1d–f ). When light at optical frequencies is scattered by a spherical nanoscale lens, it exhibits curvilinear trajectories, resulting in remarkably strong near-field magnification that produces a photonic nanojet [31] , [32] , [33] . As such, complementary to light-blocking metallic nanowire motors, self-propelled Janus spherical motors can be used as motile optical lenses to effectively concentrate the processing light and harness near-field optical effects for direct writing. Such near-field magnification leads to the creation of features with resolution beyond the diffraction limit. The Janus motors are prepared by coating transparent polystyrene or silica spheres with a thin hemispherical platinum layer for catalytic propulsion in H 2 O 2 solution. FDTD simulations provided evidence that a half-coated Janus microsphere ( Fig. 1e ) can still generate a narrow, high-intensity, subdiffraction-waist beam that propagates into the background medium. This effect is illustrated by the nanoholes obtained using stationary Janus motors as near-field lenses ( Supplementary Fig. 2 ). The simultaneous movement and light-focusing abilities of Janus sphere motors allow for the rapid and controlled transfer of the nanomotor trajectory to distinct sub-micron features in aqueous environments. Figure 1f displays a trench line created by such movement of a 2.16-μm-diameter Janus sphere motor on a positive photoresist. The FWHM of this trench is only 420 nm, which is significantly smaller than the size of the Janus motor, reflecting the effective light-focusing effect of such microspheres. Patterning by metallic nanowire motors The versatility of nanomotors gives NML the freedom for varying a wide range of experimental parameters for creating a myriad of distinct nanopatterned features. For example, the size of the nanowire motor mask can be tailored using membrane templates with different pore sizes. Here nanomotors with diameters of 200, 400 and 1000, nm were prepared for use as swimming nanomasks ( Fig. 2a–c ). The AFM images of Fig. 2d–f illustrate the morphologies of ridge lines obtained using self-propelled nanowire motors of the above diameters. As expected, nanomotor masks with smaller diameters result in higher resolution patterns, as indicated from the changes in the corresponding feature height and width. The slightly larger feature size (compared with the diameter of the swimming nanomask) is attributed to increased Brownian motion and light scattering. While these effects could compromise the positional accuracy and light masking ability for smaller motors, the FWHM of the lines drawn by 200-nm nanomotors is still in the sub-wavelength regime. An investigation of ridge-line profiles from motors with various propulsion velocities indicates that the height of the ridge decreases with increasing motor speed; intuitively, slower swimming speeds result in longer light-blocking times over their moving path ( Fig. 2g ). Meanwhile, the FWHM decreases slightly for faster motors due to the weaker influence of the Brownian motion ( Fig. 2h ). These results indicate that using nanomotors with smaller dimensions leads to an increased patterning resolution due to the nanomask shadowing effects. The resolution can also be slightly improved by increasing the motor speed, due to the reduced exposure time and influence of Brownian motion. FDTD simulations indicate that the resolution could be enhanced further by adopting a ultraviolet laser with a shorter wavelength than that of the ultraviolet lamp used here (350–450 nm). 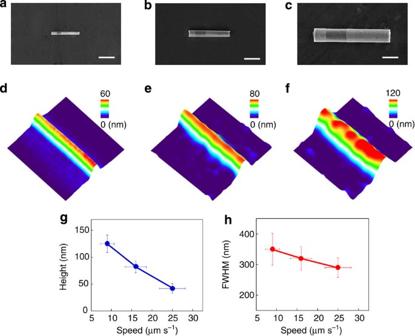Figure 2: Patterning by nanowire motors. Scanning electron microscope (SEM) images illustrating the nanowire motors with diameters of (a) 200 nm, (b) 400 nm and (c) 1000, nm. Scale bar, 1000, nm. AFM images of topographical three-dimensional (3D) line morphologies generated by nanowire motors with diameters of (d) 200 nm, (e) 400 nm and (f) 1000, nm and speed of 15 μm s−1. The 3D AFM images ind–fare shown with displayed areas of 3 × 3 μm2. Maximum height (g) and FWHM (h) of a number of single lines ‘drawn’ by the nanowire motors swimming at different speeds obtained using H2O2concentrations of 0.25, 1 and 5%. Vertical error bars represent 1 s.d. in the pattern height or FWHM (N=20). Horizontal error bars represent one s.d. in the nanomotor movement speed at the fixed fuel concentration (N=20). Figure 2: Patterning by nanowire motors. Scanning electron microscope (SEM) images illustrating the nanowire motors with diameters of ( a ) 200 nm, ( b ) 400 nm and ( c ) 1000, nm. Scale bar, 1000, nm. AFM images of topographical three-dimensional (3D) line morphologies generated by nanowire motors with diameters of ( d ) 200 nm, ( e ) 400 nm and ( f ) 1000, nm and speed of 15 μm s −1 . The 3D AFM images in d – f are shown with displayed areas of 3 × 3 μm 2 . Maximum height ( g ) and FWHM ( h ) of a number of single lines ‘drawn’ by the nanowire motors swimming at different speeds obtained using H 2 O 2 concentrations of 0.25, 1 and 5%. Vertical error bars represent 1 s.d. in the pattern height or FWHM ( N =20). Horizontal error bars represent one s.d. in the nanomotor movement speed at the fixed fuel concentration ( N =20). Full size image Remote magnetically guided writing Directional magnetic orientation of the nanowire motors can be achieved by incorporating a ferromagnetic Ni segment into the motor structure. Supplementary Movie 1 displays real-time remote magnetic control of a single nanowire motor and of two motors moving in parallel. Precise control of the nanomotor paths allows for the rapid prototyping of their trajectories to predefined patterns. 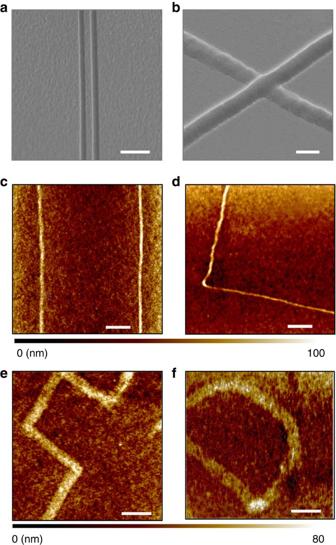Figure 3: Remote magnetically guided writing. (a) SEM images of two ridge lines generated from parallel (magnetically guidedmagnetically guided) motion of two individual nanowire motors. Diameter of nanowire motor, 400 nm. (b) Two crossed ridge lines produced from two individual staggered nanomotors under an external magnetic field. The second line resulted from the path of one nanomotor crossing over the path of another motor after turning the magnetic field. AFM images of parallel ridge lines (c) and of a right angle ridge pattern (d) generated from a longer exposure period. AFM images of a square-wave (e) and the letter ‘D’ (f) patterns obtained using moving nanomotors. Hydrogen peroxide concentration: 1%. Scale bars,a=5 μm,b=1 μm,c,d=10 μm,e,f=2 μm. Figure 3a displays a double-ridge-line feature fabricated by the simultaneous lateral movement of two individual nanomotors along the applied magnetic field. This feature illustrates the uniformity and highly parallel capabilities of the controlled nanomotor patterning concept. Figure 3b displays two crossed lines obtained as a result of one nanomotor crossing over the path of another one after turning the magnetic field. Details of the approach used for patterning such crossing features are displayed in Supplementary Fig. 3 . This illustrates the potential of using multiple motors to generate complex patterns through superposition of different motor paths. Figure 3c,d displays surface features of parallel lines and a 90-degree turn, respectively, over large areas (60 × 60 μm 2 ). Note that the length scale of the patterned lines in Fig. 3c–d is over 20 times longer than the length of the nanomotors, illustrating the capability for large-scale well-defined spatial control of the nanomotors. Figure 3e,f display a square-wave pulse pattern and a letter ‘D’ pattern, respectively. Such ability to execute discrete and continuous turns through an external magnetic field enables the patterning of both sharp vertices and smooth curves, thus leading to a wide variety of possible surface features. In addition, the magnetic field and trajectory of the nanomotors can be controlled and pre-programmed, allowing for the automatic patterning of substrates by identical motor movements. Figure 3: Remote magnetically guided writing. ( a ) SEM images of two ridge lines generated from parallel (magnetically guidedmagnetically guided) motion of two individual nanowire motors. Diameter of nanowire motor, 400 nm. ( b ) Two crossed ridge lines produced from two individual staggered nanomotors under an external magnetic field. The second line resulted from the path of one nanomotor crossing over the path of another motor after turning the magnetic field. AFM images of parallel ridge lines ( c ) and of a right angle ridge pattern ( d ) generated from a longer exposure period. AFM images of a square-wave ( e ) and the letter ‘D’ ( f ) patterns obtained using moving nanomotors. Hydrogen peroxide concentration: 1%. Scale bars, a =5 μm, b =1 μm, c , d =10 μm, e , f =2 μm. Full size image Patterning by Janus sphere motors Janus microsphere motors, which are half-coated with a Pt layer, move autonomously in a hydrogen peroxide fuel solution due to the catalytic fuel decomposition reaction [34] . When the photoresist surface is exposed to ultraviolet light, the Janus sphere motor acts as a near-field lens for nanopatterning ( Fig. 4a ). While the processing ultraviolet light illuminates a large area, it reaches a much higher intensity for photoresist exposure directly beneath the microsphere lens. The Janus sphere motors with diameter of 2.16 μm can move stably at a fixed height above the photoresist surface for uniform and consistent patterning ( Supplementary Fig. 4 ). Calculations of nanomotor–substrate distances and related information are included in the Supplementary Notes . Due to their catalytic hemispheric patch, Janus microsphere motors can lead to unique and complex optical effects unavailable for bare spheres. By carefully tuning the thickness of the platinum patch, we demonstrate that the optical properties of these motors can be intrinsically tailored from near-transparent nano-lenses to semi-opaque nanomasks, thus offering further possibilities for engineering the topography of the patterned surface features. A FDTD two-dimensional model ( Fig. 4b–d ) was used to predict how the incident light is manipulated by the engineered Janus spheres with Pt patches of different thicknesses: (b) 5 nm, (c) 40 nm and (d) 120 nm. It can be observed that the peak intensity of the photonic nanojet diminishes slightly upon increasing the Pt thickness while the opposite hemisphere remains transparent. Solvent-mediated electrostatic repulsions between the charged surfaces of the sphere and the substrate balance with van der Waals forces, resulting in an equilibrium sphere–substrate spacing, as illustrated in Supplementary Figs 5 and 6 (ref. 17 ). Very small Janus spheres (<500 nm in diameter) experience a much stronger Brownian motion that can cause fluctuations in their vertical distance from the substrate and influence the resulting patterns. Accordingly, we focus on the 4.74-μm Janus sphere motors, which always remain close to the surface and move stably at a fixed plane. The AFM images of Fig. 4e–g illustrate the ability to tailor the morphology of the generated features using Janus spheres with Pt films of different thicknesses, while Fig. 4h–j displays the corresponding cross-section profiles. The 5-nm thin Pt coating displays minimal attenuation of the incident light and thus exhibits a lower influence on the sphere’s near-field focusing, resulting in a trench line pattern ( Fig. 4e ). Note that a wider raised area surrounding the trench line was formed simultaneously as a result of light-blocking effects from the Pt patch. Increasing the thickness of the Pt film to 40 nm results in surface features of multiple symmetric ridges ( Fig. 4f ), reflecting the varied intensities of the scattered light. Further increasing the film thickness to 120 nm leads to a single ridge, consistent with results expected from an opaque mask ( Fig. 4g ). The height of the ridge line can reach 200 nm, which is comparable to heights obtained with nanowire motors. Nanopatterns with improved aspect ratio are expected by increasing the exposure dose through a higher light intensity. This versatility of Janus motors, through control of the thickness of the catalytic layer, greatly enhances the patterning capability and leads to the creation of a wide variety of distinct surface features. Further studies will focus on exploring even more complex high-aspect ratio surface patterns by changing the geometry and coverage of the Pt catalytic patch. 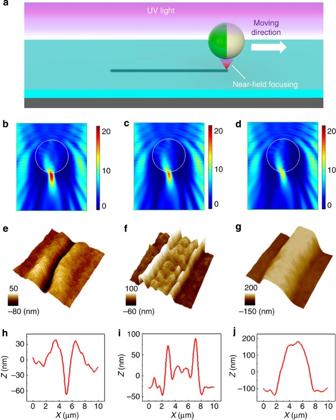Figure 4: Patterning by Janus sphere motors. (a) Schematic showing a moving Janus microsphere motor near the photoresist surface under exposure to ultraviolet light. Two-dimensional (2D) plots of the steady-state intensity of light passing through a 4.74-μm-diameter Janus sphere (silican=1.55) with Pt thickness of (b) 5 nm, (c) 40 nm and (d) 120 nm in water (n=1.34). The circle represents the contour of the sphere and the right hemisphere is coated with a Pt film. Surface morphologies and corresponding cross-section profile of the created features by using 4.74-μm Janus spheres, coated with Pt films of different thicknesses: (e) 5 nm, (f) 40 nm and (g) 120 nm. The 3D AFM images ine–gare shown with displayed areas of 10 × 10 μm2. (h–j) Representative cross-section profiles of images (d–f), respectively. Figure 4: Patterning by Janus sphere motors. ( a ) Schematic showing a moving Janus microsphere motor near the photoresist surface under exposure to ultraviolet light. Two-dimensional (2D) plots of the steady-state intensity of light passing through a 4.74-μm-diameter Janus sphere (silica n =1.55) with Pt thickness of ( b ) 5 nm, ( c ) 40 nm and ( d ) 120 nm in water ( n =1.34). The circle represents the contour of the sphere and the right hemisphere is coated with a Pt film. Surface morphologies and corresponding cross-section profile of the created features by using 4.74-μm Janus spheres, coated with Pt films of different thicknesses: ( e ) 5 nm, ( f ) 40 nm and ( g ) 120 nm. The 3D AFM images in e – g are shown with displayed areas of 10 × 10 μm 2 . ( h – j ) Representative cross-section profiles of images ( d – f ), respectively. Full size image Meanwhile, the integration of a ferromagnetic Ni layer in the Janus sphere motor can facilitate remote magnetic control for predefined writing. As illustrated in Fig. 5a , the Janus motors align such that the Janus boundary is perpendicular to the applied magnetic field, allowing for a magnetically guided patterning illustrated from AFM images of Fig. 5b,c . Under an optical microscope, the Janus boundaries of the motors are clearly and consistently observed when they are moving, indicating that the orientation of such nanolenses is preserved. Using assemblies and arrays of dynamic patterning tools is a promising pathway for the parallel fabrication of complex devices consisting of many small components. Although a variety of complex configurations are possible for assembled Janus particles, we focus here on the ‘side-by-side’ paradigmatic case to illustrate the patterning capability of such assemblies. The autonomous propulsion of different Janus motor assemblies is shown in Supplementary Movie 2 . 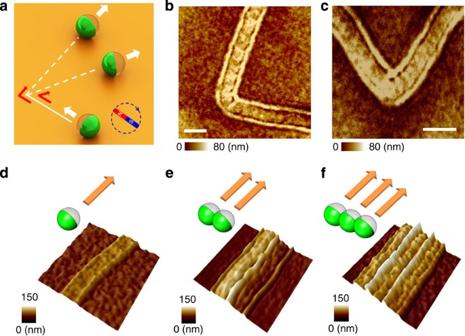Figure 5: Controlled and parallel patterning by Janus sphere motors. (a) Illustration of the magnetic guidance of Janus sphere motion. (b) A pattern created by turning the magnetic field by 90°. (c) A pattern created by turning the magnetic field by 120°. Scale bars,b–c=5 μm. Continuous patterns obtained by using (d) single, (e) double and (f) triple Janus spheres moving alongside under magnetic guidance. The three-dimensional AFM images ind–fare shown with displayed areas of 20 × 20 μm2. Figure 5d–f displays the continuous patterns obtained by such singlet, doublet and triplet Janus-sphere assemblies moving together under magnetic guidance. The various peaks in the pattern correspond to the optical field from individual Janus spheres, overlapping with each other and superimposing to form higher ridge features. These data indicate that further improvements in the pattern complexity are possible via advanced self-assembly protocols [34] , [35] , and that the diversity of the patterned features can be increased by tailoring the patch morphology of the individual Janus motors in the assembly. Figure 5: Controlled and parallel patterning by Janus sphere motors. ( a ) Illustration of the magnetic guidance of Janus sphere motion. ( b ) A pattern created by turning the magnetic field by 90°. ( c ) A pattern created by turning the magnetic field by 120°. Scale bars, b – c =5 μm. Continuous patterns obtained by using ( d ) single, ( e ) double and ( f ) triple Janus spheres moving alongside under magnetic guidance. The three-dimensional AFM images in d – f are shown with displayed areas of 20 × 20 μm 2 . Full size image We have introduced a simple and efficient nanomotor-based nano-patterning technique based on self-propelled nanomasks and nanolenses that brings a twist to conventional static optical fabrication systems. This nanomotor-fabrication strategy combines controlled movement with unique light focusing or blocking abilities for direct surface writing and provides researchers with considerable freedom for creating diverse features with different shapes and sizes. Spatially defined surface patterns, corresponding to the predetermined path of the nanomotors, can thus been generated. We expect that directional propulsion and variation of nanomotor parameters can be used to generate more elaborate functional features. For example, the shape and the number of the catalytic patches of the microsphere lenses can be customized to further increase the pattern complexity. Higher order motor organization and modular motor design should lead to further improvements in pattern intricacy. Diverse pattern morphologies can thus be achieved by rationally designing each component in the Janus motor assembly. As proof-of-concept, we demonstrate here that such nanomachines can effectively manipulate the processing light beams for optical-based nanopatterning. Future research and development of the nanomotor patterning method can be realized by combining advanced nanomotor designs with diverse functionalities. For example, it could be possible to use thermal, mechanical, electrical, plasmonic, and chemical effects for such dynamic nanomotor lithographic techniques by incorporating specific physical functionality or surface chemistry into the nanomotor. These current capabilities and future possibilities offered by motile optically active nanomachines lead to the new ‘on-the-fly’ nanomanufacturing platform and create new opportunities for surface science. Synthesis of magnetic-guided catalytic nanomotors The magnetic-guided catalytic nanomotors composed of Au, Ni, Au and Pt segments were prepared by electrodepositing the corresponding metals into 200 nm alumina membrane template (Catalogue no. 6809-6022; Whatman, Maidstone, UK) and 400 nm and 1 μm polycarbonate (PC) membrane template (Catalogue no. 800282 and 7060-2510; Whatman, New Jersey, USA). A thin silver film was first sputtered on the branched side of the alumina membrane or back side of the PC membrane to serve as a working electrode. The membrane was assembled in a plating cell with aluminium foil serving as an electrical contact for the subsequent electrodeposition. For 200 nm alumina membrane template, a sacrificial silver layer was electrodeposited into the branched area of the membrane using a silver plating solution (1025 RTU@4.5 Troy per Gallon; Technic Inc., Anaheim, CA, USA) and a total charge of 3.0 C at −0.90 V (versus Ag/AgCl, in connection to a Pt wire counter electrode). This was followed by an electrodeposition of gold for 0.75 C from a gold plating solution (Orotemp 24 RTU RACK; Technic Inc.) at −1.0 V. Subsequently, nickel was electrodeposited at −1.0 V from a nickel plating solution (20 g l −1 NiCl 2 ·6H 2 O, 515 g l −1 Ni(H 2 NSO 3 ) 2 ·4H 2 O, and 20 g l −1 H 3 BO 3 ) using a total charge of 2.0 C. Another gold segment was then electrodeposited for 0.75 C, followed by the Pt segment galvanostatically deposited at −2 mA for 50 min using a platinum plating solution (Platinum RTP; Technic Inc.). For 400 nm and 1 μm PC membrane templates, a sacrificial silver layer was first electrodeposited for a total charge of 1.0 C at −0.9 V. Subsequently, gold layer was electroplated for a total charge of 0.25 C at −1.0 V, followed by nickel layer for 2 C at −1.0 V and 0.25 C of gold at −1.0 V. Finally, Pt segment was electroplated at −2 mA for 20 min. The sputtered and sacrificial silver layers were simultaneously removed by mechanical polishing using cotton tip applicators soaked with 35% HNO 3 . The alumina membrane was removed in 3 M NaOH for 30 min. The resulting nanowires were collected by centrifugation at 7,000 r.p.m. for 5 min and washed repeatedly with deionized water until a neutral pH was achieved. The PC membrane was removed in methylene chloride for 5 min to completely release the nanowires. The corresponding nanowires were collected by centrifugation at 6,000 r.p.m. for 1 min and washed repeatedly with methylene chloride, followed by ethanol (two times) and ultrapure water (three times). Synthesis of Janus micromotors The Janus micromotors were prepared using silica microspheres (1.21 and 4.74 μm mean diameter, Bangs Laboratories, Fishers, IN, USA) and polystyrene microspheres (0.72 and 2.16 μm mean diameter, Bangs Laboratories) as the base particles. Twenty microlitres of microspheres solution was first dispersed into water and centrifuged. Then, the microspheres were redispersed in 200 μl water. The sample was then spread onto glass slides and dried uniformly to form microsphere monolayers. These spheres were closely packed in contact with each other due to the van der Waals forces. The microspheres were sputter coated with a 10 nm Pt layer using a Denton Discovery 18 sputtering system. The deposition was performed at room temperature with a DC power of 200 W and Ar pressure of 2.5 mT for 10 s. To ensure a uniform Janus half-shell coating, the substrate rotation speed was set as 0 and the sample slides were set up at an angle parallel to the Pt target. Subsequently, the Janus particles were detached from the substrate via sonication or pipette pumping and were dispersed in water again to form the micromotor solution. The singlet Janus motors were obtained by a long sonication time (>1 min), while doublet and triplet Janus motors were created using significantly shorter sonication periods (~5 s). Lithography process The photoresist (MicroPosit SC-1827) was spin-coated onto a silicon wafer at 3,000 r.p.m. for 40 s. The wafer was prebaked for 1 min at 115 °C. A 20 μl drop of nanomotor solution was placed on the coated photoresist followed by a 20 μl drop of hydrogen peroxide fuel (with concentrations varying from 0.25 to 10%). The sample cell was then translated to a Karl Suss MA6 Mask Aligner (wavelength range UV400 350–450 nm, Power 11 mW cm −2 ). The exposure time varied from 2 to 16 s, depending upon the predefined pattern. A neodymium magnet was used for the remote magnetic guidance during exposure. After exposure, the solution on the photoresist was removed by water rinsing and the sample was developed in MF-321. Equipment Template electrochemical deposition of the micromotors was carried out with a CHI 660D potentiostat (CH Instruments, Austin, TX, USA). Scanning electron microscopy (SEM) images were obtained with a Phillips XL30 ESEM instrument, using an acceleration potential of 20 kV. AFM images were taken with Veeco Scanning Probe Microscope. Videos were captured at 45 frames per second by an inverted optical microscope (Nikon Instrument Inc. Ti-S/L100), coupled with a × 40 objective Hamamatsu digital camera C11440, using the NIS-Elements AR 3.2 software. How to cite this article: Li, J. et al. Nanomotor lithography. Nat. Commun. 5:5026 doi: 10.1038/ncomms6026 (2014).